An alternate binding site for PPARγ ligands PPARγ is a target for insulin-sensitizing drugs such as glitazones, which improve plasma glucose maintenance in patients with diabetes. Synthetic ligands have been designed to mimic endogenous ligand binding to a canonical ligand-binding pocket to hyperactivate PPARγ. Here we reveal that synthetic PPARγ ligands also bind to an alternate site, leading to unique receptor conformational changes that impact coregulator binding, transactivation and target gene expression. Using structure–function studies we show that alternate site binding occurs at pharmacologically relevant ligand concentrations, and is neither blocked by covalently bound synthetic antagonists nor by endogenous ligands indicating non-overlapping binding with the canonical pocket. Alternate site binding likely contributes to PPARγ hyperactivation in vivo , perhaps explaining why PPARγ full and partial or weak agonists display similar adverse effects. These findings expand our understanding of PPARγ activation by ligands and suggest that allosteric modulators could be designed to fine tune PPARγ activity without competing with endogenous ligands. Nuclear receptors (NRs) are ligand-regulated transcription factors that function as allosteric protein scaffolds recruiting chromatin remodeling machinery to promoter regions of target genes [1] . Recent studies have explored the structural features of full-length NR complexes [2] , [3] , [4] , [5] , [6] , yet ligand-driven structural changes that are critical for determining the molecular basis for the pharmacological and functional response to ligands remain unclear. Endogenous and synthetic ligands are understood to compete for binding to an internal hydrophobic ligand-binding pocket (LBP) located within the NR ligand-binding domain (LBD). Ligands bind the LBP, which is a hydrophobic core within the 12 helix bundle LBD [7] , altering the hydrogen bond network that can stabilize a key switch helix, helix 12 (H12). In the absence of ligand, H12 is highly dynamic and in equilibrium among many conformations ranging from active to inactive. Ligand binding can stabilize the dynamics of helix 12 and alter the coregulator protein interaction surface of the LBD, which is referred to as the activation function-2 (AF-2) surface. The AF-2 surface is a three-dimensional (3D) surface that includes H3, H3-4 loop, H11 and H12. The active conformation favours coactivator binding, and when the equilibrium is shifted towards the inactive state corepressor binding is favoured. These specific interactions affect the transactivation activity of the receptor and modulate the expression of receptor target genes. Ligand-induced activation of NRs was initially viewed as a straightforward ‘on–off’ switch [8] , [9] . However, more complex mechanisms of ligand-induced regulation of NR function are becoming clear. For example, we have shown that PPARγ ligands can differentially affect the structural conformation of two distinct surfaces important to interaction with various PPARγ partners and the post-translational modification status of PPARγ [10] , [11] . We also described a dynamic mechanism by which ligand binding partially stabilizes the PPARγ AF-2 surface for partial agonist activity [12] , [13] . In addition, serotonin and fatty acid metabolites can bind simultaneously to distinct sub-regions within the PPARγ LBP, suggesting a mechanism to integrate signals from distinct signalling pathways [14] . Here we demonstrate that synthetic ligands designed to mimic the activity of endogenous ligands via binding to the canonical LBP in PPARγ can also bind to an alternate site. Alternate site binding occurs via three mechanisms of potential pharmacological relevance, including (1) binding two molar equivalents of ligand to PPARγ, one to the canonical LBP and a second to the alternate site; (2) binding when the canonical LBP is ‘blocked’ by a covalently bound irreversible antagonist; and (3) binding when the canonical LBP is covalently bound to an endogenous ligand. Alternate site binding likely contributes to the pharmacological response of PPARγ ligands, which could impact the interpretation of studies examining the function of PPARγ using synthetic ligands and opens up the possibility of fine tuning PPARγ activity with synthetic allosteric modulators in the presence of endogenous ligands. PPARγ binds two molar equivalents of synthetic ligand We used 19 F NMR to monitor the binding of two synthetic PPARγ ligands, MRL20 and MRL24 ( Fig. 1a ; compounds 20 and 24 (ref. 15 )), to PPARγ. Stoichiometric addition of MRL20 ( Fig. 1b,c and Supplementary Fig. 1 ) or MRL24 ( Fig. 1d,e ) to PPARγ reveals a sequential saturation of two 19 F NMR resonances. Population of the second MRL20 19 F NMR resonance did not decrease the peak intensity or volume of the first 19 F NMR resonance, but it caused a slight change in chemical shift and linewidth of the first 19 F NMR resonance ( ∼ 20 Hz). The canonical LBP-binding affinity of MRL20 is 2 nM (ref. 15 ). Using 19 F NMR, we calculated the binding affinity of the second MRL20 binding event to be ∼ 4 μM. These MRL20-binding affinities are confirmed by time-resolved Förster resonance energy transfer (TR-FRET) experiments below. The sequential population of two MRL20 19 F NMR resonances is consistent with two MRL20 ligands binding to PPARγ with ∼ 1,000-fold difference in binding affinity. We previously proposed that multiple MRL20 NMR resonances could correspond to a single ligand-binding event with multiple binding modes [12] , and we confirmed that this indeed occurs at 1:1 ligand:PPARγ ( Supplementary Fig. 2 ). In addition, these new data implicate a second ligand-binding event that occurs within the context of the PPARγ/RXRα LBD heterodimer ( Fig. 1f ) and full-length PPARγ ( Fig. 1g ), which is specific as no binding was observed to a control protein, lysozyme ( Fig. 1h ). 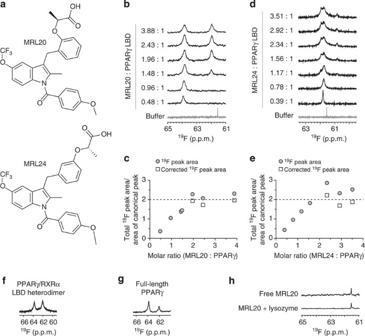Figure 1: MRL20 and MRL24 bind to PPARγwith a 2:1 stoichiometry. (a) Chemical structure of MRL20 and MRL24. Titration of (b,c) MRL20 or (d,e) MRL24 results in the population of two PPARγ LBD-bound19F NMR resonances, where (c,e) are a plot of the total19F peak area in (b) and (d), normalized to the area of the saturated canonical peak; concentrations beyond two molar equivalents of ligand are corrected (free ligand signal subtracted and adjusted for differential longitudinal relaxation; see methods for details). (f,g) MRL20 populates two19F NMR resonances within the context of the (f) PPARγ/RXRα LBD heterodimer and (g) full-length PPARγ. (h) A single, sharp19F resonance is observed for free MRL20 in buffer or added to lysozyme, indicating that alternate site binding of MRL20 to PPARγ occurs in a specific manner. Figure 1: MRL20 and MRL24 bind to PPAR γ with a 2:1 stoichiometry. ( a ) Chemical structure of MRL20 and MRL24. Titration of ( b , c ) MRL20 or ( d , e ) MRL24 results in the population of two PPARγ LBD-bound 19 F NMR resonances, where ( c , e ) are a plot of the total 19 F peak area in ( b ) and ( d ), normalized to the area of the saturated canonical peak; concentrations beyond two molar equivalents of ligand are corrected (free ligand signal subtracted and adjusted for differential longitudinal relaxation; see methods for details). ( f , g ) MRL20 populates two 19 F NMR resonances within the context of the ( f ) PPARγ/RXRα LBD heterodimer and ( g ) full-length PPARγ. ( h ) A single, sharp 19 F resonance is observed for free MRL20 in buffer or added to lysozyme, indicating that alternate site binding of MRL20 to PPARγ occurs in a specific manner. Full size image Structural mapping of the alternate binding site in PPARγ We performed a series of 2D [ 1 H, 15 N]-TROSY-HSQC NMR experiments to map the effect of the second ligand-binding event. Using additional NMR data and other assignments [16] , we extended PPARγ NMR chemical shift assignments for MRL20 and MRL24 (ref. 12 ) in the following regions: H2′–H3, β-sheet region and loops, the Ω loop (a flexible loop region comprising ∼ 15 residues between H2′ and H3 spanning D260-K275), H11 and H12. Titration of MRL20 up to 1:1 (ligand:protein) reveals a transition in slow exchange on the NMR timescale ( Fig. 2a ), indicating a high-affinity binding event consistent with a 2 nM LBP affinity [15] . Higher stoichiometries reveal a second transition where some peaks are affected by subtle chemical shift changes and line broadening, consistent with exchange effects expected [17] for a ligand with ∼ 4 μM binding affinity. 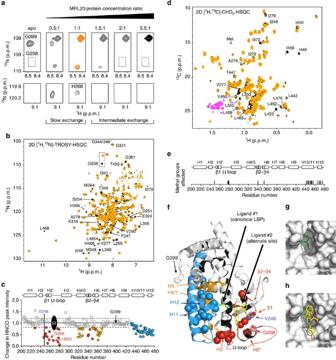Figure 2: Mapping the alternate MRL20 binding site in PPARγ. (a) Titration of MRL20 into15N-PPARγ LBD monitored by 2D [1H,15N]-TROSY-HSQC NMR reveals two binding transitions. The first slow exchange transition corresponds to the canonical LBP binding event (apo to 1:1), and the second intermediate exchange transition to the alternate site binding event (>1:1 stoichiometry). (b) Comparison of 2D [1H,15N]-TROSY-HSQC spectra for15N-PPARγ LBD bound to one or two molecules of MRL20 (black and orange, respectively). (c) NMR chemical shift footprinting reveals a decrease in peak intensity between 3D TROSY-HNCO experiments collected for2H,13C,15N-PPARγ LBD bound to one or two molecules of MRL20 (black/pink and orange/grey, respectively, for positive/negative peak amplitudes) and reveals residues affected by the alternate site-binding event. (d) Comparison of 2D [1H,13C]-methyl CHD2-detected HSQC data for2H,13C,15N-PPARγ LBD bound to one or two molecules of MRL20. (e) Residues with methyl NMR resonances affected upon binding a second MRL20 ligand. (f) NMR chemical shift footprinting changes mapped onto the PPARγ LBD structure reveals the site of interaction (red) and regions allosterically affected by alternate site binding (blue, orange); spheres represent methyl groups affected, and regions coloured black have unassigned NMR chemical shifts likely due to dynamics on the NMR intermediate exchange regime; the dynamic Ω loop, which comprises part of the alternate site, is illustrated with a dotted line. (g) The alternate site is formed by a solvent-accessible pocket on the PPARγ LBD surface. (h) Molecular docking of a second MRL20 ligand (yellow) into the alternate site, which is also shown in (f). Figure 2: Mapping the alternate MRL20 binding site in PPAR γ . ( a ) Titration of MRL20 into 15 N-PPARγ LBD monitored by 2D [ 1 H, 15 N]-TROSY-HSQC NMR reveals two binding transitions. The first slow exchange transition corresponds to the canonical LBP binding event (apo to 1:1), and the second intermediate exchange transition to the alternate site binding event (>1:1 stoichiometry). ( b ) Comparison of 2D [ 1 H, 15 N]-TROSY-HSQC spectra for 15 N-PPARγ LBD bound to one or two molecules of MRL20 (black and orange, respectively). ( c ) NMR chemical shift footprinting reveals a decrease in peak intensity between 3D TROSY-HNCO experiments collected for 2 H, 13 C, 15 N-PPARγ LBD bound to one or two molecules of MRL20 (black/pink and orange/grey, respectively, for positive/negative peak amplitudes) and reveals residues affected by the alternate site-binding event. ( d ) Comparison of 2D [ 1 H, 13 C]-methyl CHD 2 -detected HSQC data for 2 H, 13 C, 15 N-PPARγ LBD bound to one or two molecules of MRL20. ( e ) Residues with methyl NMR resonances affected upon binding a second MRL20 ligand. ( f ) NMR chemical shift footprinting changes mapped onto the PPARγ LBD structure reveals the site of interaction (red) and regions allosterically affected by alternate site binding (blue, orange); spheres represent methyl groups affected, and regions coloured black have unassigned NMR chemical shifts likely due to dynamics on the NMR intermediate exchange regime; the dynamic Ω loop, which comprises part of the alternate site, is illustrated with a dotted line. ( g ) The alternate site is formed by a solvent-accessible pocket on the PPARγ LBD surface. ( h ) Molecular docking of a second MRL20 ligand (yellow) into the alternate site, which is also shown in ( f ). Full size image To determine the location of the alternate ligand-binding site, we compared NMR peak intensities for backbone NH groups in 2D [ 1 H, 15 N]-TROSY-HSQC ( Fig. 2b ) and 3D TROSY-HNCO ( Fig. 2c ), and methyl groups in 2D [ 1 H, 13 C]-CHD 2 -HSQC ( Fig. 2d,e ) data for PPARγ bound to one or two molecules of MRL20. The most significant drop in HNCO peak intensity occurs for residues in β-strand 1 (β1), H2′, the Ω loop, β2-4 and the surrounding loops ( Fig. 2f ; red and purple), indicating this is likely the alternate binding site for the second MRL20 ligand. A pocket is present at this site ( Fig. 2g ) posited to be the ligand entry/exit site to the canonical LBP [18] , [19] . Molecular docking demonstrates a second MRL20 molecule can bind to this pocket ( Fig. 2h ), which is bound on one side by the Ω loop—a flexible loop region between H2′ and H3 in the LBD that is commonly unobserved in crystal structures due to its high mobility. This alternate ligand-binding site encompasses an area not thought of as part of the canonical LBP. Several other regions distant from this alternate binding site display a notable decrease in NMR peak intensity ( Fig. 2f ; orange and blue), though not as significant as the alternate site, including the AF-2 surface. MRL24 induces similar alternate site-binding effects ( Fig. 3 ). These data implicate an allosteric structural coupling between alternate site binding and the AF-2 coregulator-binding surface. 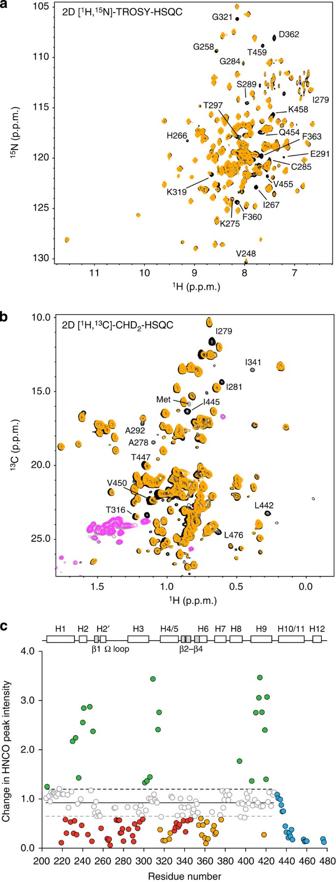Figure 3: Mapping the alternate MRL24-binding site in PPARγ. (a) Comparison of 2D [1H,15N]-TROSY-HSQC spectra for15N-PPARγ LBD bound to one or two molecules of MRL24 (black and orange, respectively). (b) Comparison of 2D [1H,13C]-methyl CHD2-detected HSQC data for2H,13C,15N-PPARγ LBD bound to one or two molecules of MRL24. (c) NMR chemical shift footprinting reveals a decrease in peak intensity between 3D TROSY-HNCO experiments collected for2H,13C,15N-PPARγ LBD bound to one or two molecules of MRL24 (black/pink and orange/grey, respectively, for positive/negative peak amplitudes) and reveals residues affected by the alternate site-binding event. Figure 3: Mapping the alternate MRL24-binding site in PPAR γ . ( a ) Comparison of 2D [ 1 H, 15 N]-TROSY-HSQC spectra for 15 N-PPARγ LBD bound to one or two molecules of MRL24 (black and orange, respectively). ( b ) Comparison of 2D [ 1 H, 13 C]-methyl CHD 2 -detected HSQC data for 2 H, 13 C, 15 N-PPARγ LBD bound to one or two molecules of MRL24. ( c ) NMR chemical shift footprinting reveals a decrease in peak intensity between 3D TROSY-HNCO experiments collected for 2 H, 13 C, 15 N-PPARγ LBD bound to one or two molecules of MRL24 (black/pink and orange/grey, respectively, for positive/negative peak amplitudes) and reveals residues affected by the alternate site-binding event. Full size image Covalent antagonists do not block alternate site binding GW9662 and T0070907 ( Fig. 4a ) are synthetic irreversible PPARγ antagonists that covalently attach to Cys285 (refs 20 , 21 , which points into the PPARγ LBP ( Fig. 4b ). Covalent antagonists block binding of other ligands to the LBP ( Fig. 4c ), and because they are thought to completely block ligand binding to PPARγ they are used as chemical tools to determine whether or not ligand binding to PPARγ is involved in a particular functional response. If another PPARγ ligand shows activity when coadministered with a covalent antagonist, the ligand is said to have PPARγ-independent, or off-target, functional effects. Analysis of the GW9662-PPARγ co-crystal structure suggested that GW9662 or T0070907 would block MRL20 binding to the canonical LBP but not the alternate site. To test this we exposed PPARγ to GW9662 or T0070907, added a saturating amount of MRL20 and performed 19 F NMR. MRL20 ( Fig. 4d ) or MRL24 ( Fig. 4e ) binding to PPARγ covalently bound to an antagonist populates a single 19 F NMR resonance. This effect is dependent on Cys285, as pretreatment of a Cys285Ala mutant with covalent antagonist shows two peaks when saturated with MRL20. The MRL20 19 F chemical shift in the presence of GW9662 (61.95 p.p.m.) and T0070907 (62.55 p.p.m.) is similar to the chemical shift of the second MRL20 ( Fig. 1b ) that binds to the alternate site (62.1 p.p.m. ), indicating they likely bind within the same alternate site. The only difference between GW9662 and T0070907 is a single nitrogen substitution ( Fig. 4a ). Thus, the different alternate-site-bound 19 F chemical shifts for MRL20 bound to GW9662-PPARγ versus T0070907-PPARγ suggest that these antagonists are in close structural proximity to MRL20 bound to the alternate -site, which is consistent with a docking model ( Fig. 4f ). 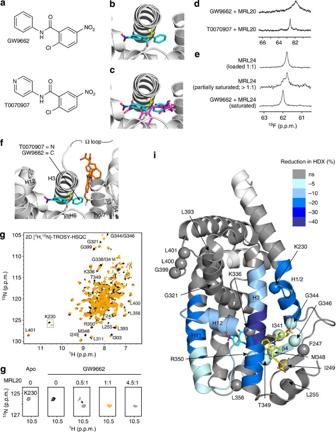Figure 4: Covalent antagonists do not block alternate site ligand binding to PPARγ. (a) Chemical structures of GW9662 and T0070907. (b) GW9662 (cyan) covalently attaches to PPARγ residue C285 (yellow). (c) When GW9662 (cyan) is covalently bound to PPARγ, it sterically blocks MRL20 (magenta) from binding to the LBP. (d,e)19F NMR reveals (d) MRL20 and (e) MRL24 bind to PPARγ LBD bound to a covalent antagonist and populate a single resonance. (f) Molecular docking of MRL20 ligand into the alternate site of PPARγ LBD covalently bound to GW9662. (g) 2D [1H,15N]-TROSY-HSQC NMR confirms that MRL20 binds to15N-PPARγ LBD covalently bound to GW9662. (h) Titration of MRL20 into GW9662-bound15N-PPARγ LBD monitored by 2D [1H,15N]-TROSY-HSQC NMR reveals MRL20 binding effects occurring in slow exchange at residues remote from the alternate binding site. (i) HDX-MS analysis reveals that alternate site binding of MRL20 to PPARγ LBD covalently bound to GW9962 causes protection from HDX in the alternate site region and the PPARγ AF-2 surface. Figure 4: Covalent antagonists do not block alternate site ligand binding to PPAR γ . ( a ) Chemical structures of GW9662 and T0070907. ( b ) GW9662 (cyan) covalently attaches to PPARγ residue C285 (yellow). ( c ) When GW9662 (cyan) is covalently bound to PPARγ, it sterically blocks MRL20 (magenta) from binding to the LBP. ( d , e ) 19 F NMR reveals ( d ) MRL20 and ( e ) MRL24 bind to PPARγ LBD bound to a covalent antagonist and populate a single resonance. ( f ) Molecular docking of MRL20 ligand into the alternate site of PPARγ LBD covalently bound to GW9662. ( g ) 2D [ 1 H, 15 N]-TROSY-HSQC NMR confirms that MRL20 binds to 15 N-PPARγ LBD covalently bound to GW9662. ( h ) Titration of MRL20 into GW9662-bound 15 N-PPARγ LBD monitored by 2D [ 1 H, 15 N]-TROSY-HSQC NMR reveals MRL20 binding effects occurring in slow exchange at residues remote from the alternate binding site. ( i ) HDX-MS analysis reveals that alternate site binding of MRL20 to PPARγ LBD covalently bound to GW9962 causes protection from HDX in the alternate site region and the PPARγ AF-2 surface. Full size image We confirmed that MRL20 binds to GW9662-PPARγ LBD using 2D [ 1 H, 15 N]-TROSY-HSQC NMR ( Fig. 4g ). MRL20 binding to the alternate site of GW9662-PPARγ causes line broadening and chemical shift perturbations for residues within the vicinity of the alternate site and the AF-2 surface. Although alternate site binding of MRL20 to GW9662-PPARγ causes substantial line broadening for residues within the alternate site, other resonances distant from this alternate site display a transition in slow exchange on the NMR timescale ( Fig. 4h ). An interpretation of the mixed intermediate/slow exchange effects is that the binding affinity of MRL20 for the alternate site is higher when the LBP is blocked with GW9662 compared with when the LBP is occupied by MRL20. This is confirmed by TR-FRET measurement below. However, despite the higher alternate site affinity, the 19 F NMR resonance for MRL20 bound to the alternate site is broader when bound to GW9662-PPARγ ( Fig. 4d ) compared with MRL20-bound PPARγ ( Fig. 1b ). This indicates a large degree of conformational heterogeneity when bound to the alternate site of GW9662-PPARγ, such as multiple binding modes [22] or motion/exchange on the μs–ms timescale [17] , providing an explanation for the intermediate exchange observed for residues near the alternate site. Alternate site binding stabilizes the AF-2 surface These NMR data demonstrate that covalent antagonists block binding of MRL20 to the canonical PPARγ LBP but not the alternate site, which we confirmed using molecular docking ( Fig. 4f ). Thus, treatment of PPARγ with these covalent antagonists allows the study of alternate site binding specifically on the structure and function of PPARγ. Approximately half of the NMR resonances are missing in GW9662–PPARγ ( Supplementary Fig. 3 ). We therefore used hydrogen/deuterium exchange (HDX) mass spectrometry (MS) to monitor changes in solvent accessibility and hydrogen bonding caused by binding of MRL20 to the alternate site of GW9662–PPARγ. Incubation of PPARγ with GW9662 resulted in a mass shift of the H3 peptide containing Cys285 by +241.062 Da. We were unable to detect unmodified H3 peptide confirming complete covalent attachment of GW9662 to PPARγ. MRL20 induced robust protection from HDX in GW9662-PPARγ within several structural regions ( Fig. 4i and Supplementary Table 1 ) including the alternate site and the AF-2 surface. Qualitatively, the pattern of HDX protection on the AF-2 surface caused by alternate site binding of MRL20 to GW9662-PPARγ is similar to what we observed previously for MRL20 binding to the canonical LBP using a 10 × molar excess of ligand [12] , [13] . One exception is a peptide from H6/7, which is protected upon binding MRL20 to the LBP but not to the alternate site of GW9662-PPARγ. This peptide is in close proximity to the canonical LBP-bound MRL20 but not the alternate site, possibly explaining why it is not affected by alternate site binding of MRL20 to GW9662–PPARγ. Alternate site binding affects coregulator interaction To determine whether alternate site ligand binding can affect the interaction between coregulator proteins and PPARγ, we performed a TR-FRET assay to monitor the ability of ligands to affect coregulator peptide binding to the PPARγ LBD. MRL20 causes a concentration-dependent increase in association between a peptide fragment ‘NR box’ of the TRAP220 coactivator (13 nM EC 50 ) ( Fig. 5a,b ). Furthermore, there is a subtle but notable effect on TRAP220 binding around the expected alternate site K d ( ∼ 2 μM; Fig. 5c ). MRL20 binding to the alternate site of GW9662–PPARγ and T0070907–PPARg causes a potent and robust increase in TRAP220 binding (361 nM and 2 μM EC 50 , respectively), indicating the phenyl (GW9662) to pyridyl (T0070907) group modification affects alternate site-binding affinity. Antagonist treatment of a Cys285Ala mutant does not affect MRL20 EC 50 values, confirming that covalent attachment to Cys285 is necessary for the right-shifted EC 50 values ( Fig. 5d ). In addition, the alternate site response occurs for full-length PPARγ with and without its heterodimer partner, RXRα ( Fig. 5e ). 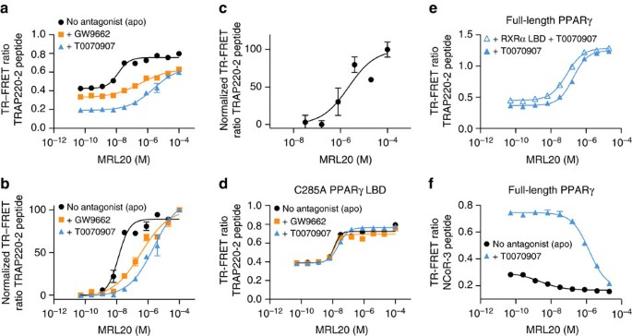Figure 5: Alternate site binding affects PPARγ–coregulator interaction. (a) TR-FRET assay showing the effect of MRL20 on TRAP220-2 peptide binding to PPARγ protein in the absence or presence of a covalent antagonist, performed in duplicate and plotted as the average (±s.d.). (b) Same data as (a) but normalized to illustrate the biphasic response for MRL20 to apo PPARγ and the EC50differences between all conditions. (c) Same as in (b) but focused on the alternate site response for apo PPARγ. (d) PPARγ C285A mutation serves as a control to show that C285 is critical for covalent antagonist attachment and blocking MRL20 binding to the LBP in the TR-FRET assay. (e,f) TR-FRET assay shows an alternate-site response for MRL20 using (e) full-length PPARγ protein and full-length PPARγ protein heterodimerized to RXRα LBD covalently bound to T0070907 performed in duplicate and plotted as the average (±s.d.). (f) Covalent attachment of T0070907 increases the basal interaction of NCoR-3 peptide right shifts the MRL20 IC50compared with apo PPARγ, performed in duplicate and plotted as the average (±s.d.). All data fit to a sigmoidal dose response curve. Figure 5: Alternate site binding affects PPAR γ –coregulator interaction. ( a ) TR-FRET assay showing the effect of MRL20 on TRAP220-2 peptide binding to PPARγ protein in the absence or presence of a covalent antagonist, performed in duplicate and plotted as the average (±s.d.). ( b ) Same data as ( a ) but normalized to illustrate the biphasic response for MRL20 to apo PPARγ and the EC 50 differences between all conditions. ( c ) Same as in ( b ) but focused on the alternate site response for apo PPARγ. ( d ) PPARγ C285A mutation serves as a control to show that C285 is critical for covalent antagonist attachment and blocking MRL20 binding to the LBP in the TR-FRET assay. ( e , f ) TR-FRET assay shows an alternate-site response for MRL20 using ( e ) full-length PPARγ protein and full-length PPARγ protein heterodimerized to RXRα LBD covalently bound to T0070907 performed in duplicate and plotted as the average (±s.d.). ( f ) Covalent attachment of T0070907 increases the basal interaction of NCoR-3 peptide right shifts the MRL20 IC 50 compared with apo PPARγ, performed in duplicate and plotted as the average (±s.d.). All data fit to a sigmoidal dose response curve. Full size image Profiling a diverse set of synthetic PPARγ ligands We next determined whether functional effects of alternate site binding occur with other synthetic PPARγ ligands by monitoring NCoR or TRAP220 peptide recruitment to PPARγ as a function of ligand concentration for a diverse set of PPARγ ligands and control non-PPARγ ligands. Antagonist treatment increases NCoR recruitment ( Fig. 5f ) and decreases TRAP220 recruitment ( Fig. 5a ) compared with apo PPARγ. Most synthetic PPARγ ligands profiled display some degree of alternate site binding effects to antagonist-bound PPARγ with varying potencies ( Supplementary Fig. 4 ). Ligands that show alternate site binding effects in a saturating and concentration-dependent manner with potencies near or below 1 μM include SR9034 (65 nM; compound 7b [23] ), MRL24 (175 nM), nTZDpa (264 nM), SR1988 ( 1 ; 356 nM), SR1664 (ref. 10 ) (384 nM), SR2088 ( 2 ; 461 nM) and BVT.13 (2.44 μM). The binding modes of ligands that have published co-crystal structures overlap with that of GW9662, although for nTZDpa and BVT.13 the overlap is less severe. This implies that although these ligands do not bind to GW9662–PPARγ using the crystalized binding modes, the alternate site binding modes for these ligands have a potent functional effect. PPARγ full agonists GW1929 and thiazolidinediones (TZDs) rosiglitazone, pioglitazone, troglitazone and ciglitazone displayed less potent and/or efficacious alternate site functional effects. Two naturally occurring plant compounds reported to modulate PPARγ activity, daidzein and resveratrol, show prominent alternate site functional effects. Finally, we tested several non-PPARγ ligands, including ligands of other NRs, most of which showed no significant alternate site response. Thus, the functional response to alternate site binding is more potent and efficacious for synthetic PPARγ ligands versus non-PPARγ ligands. For some ligands, it is possible that alternate site effects in this assay could be attributed to ligand aggregation or precipitation at high concentrations. However, this does not appear to be the case at least for MRL20, MRL24 and rosiglitazone ( Supplementary Figs 5 and 6 ). Alternate site binding affects transactivation Luciferase reporter assays are used to measure NR-dependent transcription, or transactivation, in cells. In general, rosiglitazone, MRL20 and MRL24 display concentration-dependent increases in PPARγ transactivation with potencies (EC 50 ) consistent with their canonical LBP-binding affinities ( Fig. 6a ) [12] . However MRL24, a poor activator of PPARγ transcription, still shows an increase in transactivation at concentrations >200-fold higher than its 2 nM canonical LBP binding affinity [15] , indicating there may be contributions from alternate site binding. To further determine whether alternate site ligand binding can affect PPARγ transactivation, we performed a cotransfection assay by preincubating cells with GW9662 before treating cells with ligand ( Fig. 6b ). GW9662 did not block the action of MRL20 and MRL24 with EC 50 values consistent with the TR-FRET coregulator assay (317 nM and 62 nM, respectively). Also consistent with TR-FRET coregulator binding data ( Supplementary Fig. 4j ), GW9662 blocks the action of rosiglitazone at concentrations up to ∼ 2 μM, whereas higher rosiglitazone concentrations elicit an increase in PPARγ transactivation. 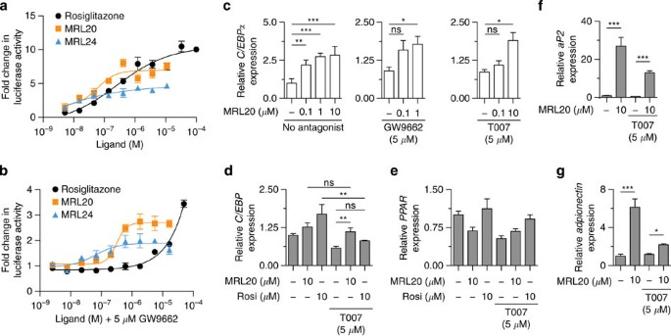Figure 6: Alternate site binding affects PPARγtransactivation and target gene expression. (a,b) Luciferase reporter assay showing the concentration-dependent effects of MRL20, MRL24 and rosiglitazone on PPARγ transactivation (a) without GW9662 pretreatment and (b) with GW9662 pretreatment, performed by cotransfection of Gal4-PPARγ LBD andUAS::lucreporter plasmid, performed in triplicate and plotted with the average (±s.e.m.) and fit to a sigmoidal dose response curve. (c) qRT–PCR analysis ofC/EBPαexpression in Jurkat cells, performed in quadruplicate, plotted with the average (±s.e.m.), and analysed using Bonferronipost hoccomparison; ns=not significant. (d–g) qRT–PCR analysis of PPARγ target genes in NIH-3T3-L1 cells harvested 3 days after inducing differentiation, performed in quadruplicate, plotted with the average (±s.e.m.), and analysed using one-way ANOVA with Tukeypost hoccomparison; ns=not significant. T007=T0070907. Figure 6: Alternate site binding affects PPAR γ transactivation and target gene expression. ( a , b ) Luciferase reporter assay showing the concentration-dependent effects of MRL20, MRL24 and rosiglitazone on PPARγ transactivation ( a ) without GW9662 pretreatment and ( b ) with GW9662 pretreatment, performed by cotransfection of Gal4-PPARγ LBD and UAS::luc reporter plasmid, performed in triplicate and plotted with the average (±s.e.m.) and fit to a sigmoidal dose response curve. ( c ) qRT–PCR analysis of C/EBPα expression in Jurkat cells, performed in quadruplicate, plotted with the average (±s.e.m. ), and analysed using Bonferroni post hoc comparison; ns=not significant. ( d – g ) qRT–PCR analysis of PPARγ target genes in NIH-3T3-L1 cells harvested 3 days after inducing differentiation, performed in quadruplicate, plotted with the average (±s.e.m. ), and analysed using one-way ANOVA with Tukey post hoc comparison; ns=not significant. T007=T0070907. Full size image Alternate site binding affects target gene expression We next assessed the effect of MRL20 binding to the alternate site of endogenous PPARγ in Jurkat T-lymphocyte cells. In the absence of covalent antagonist, MRL20 causes a concentration-dependent increase in C/EBPα expression ( Fig. 6c ). Coadministration of a covalent antagonist (GW9662 or T0070907) and MRL20 did not block the action of MRL20 on C/EBPα expression, but rather caused a right-shift in the efficacy of MRL20. Consistent with our TR-FRET data ( Fig. 5a,b ), the rank order of potency for MRL20 inducing C/EBPα expression is no covalent antagonist>GW9662>T0070907. We also assessed the action of alternate site binding in the NIH-3T3-L1 preadipocyte cell line, which is a commonly used cell model to assess endogenous PPARγ function related to adipocyte differentiation. NIH-3T3-L1 cells were differentiated in the presence of MRL20 or rosiglitazone with or without coadministered covalent antagonist and harvested 3 days after initiating differentiation. In the absence of antagonist both MRL20 and rosiglitazone increase C/EBPα expression ( Fig. 6d ). However, coadministration of T0070907 significantly reduced the efficacy of rosiglitazone, but not MRL20, on inducing C/EBPα expression. This occurs without significantly affecting PPARγ expression ( Fig. 6e ). We also tested the effect of MRL20, with and without T0070907 coadministration, on the expression of aP2 ( Fig. 6f ) and adiponectin ( Fig. 6g ), which are genes regulated by classical PPARγ-driven transcriptional agonism and phosphorylation of PPARγ, respectively [10] , [11] . MRL20 alone and MRL20 coadministered with T0070709 both significantly increased the expression of these genes. This indicates that binding of MRL20 to the alternate site can affect the activity of endogenous PPARγ in cells and that alternate site binding affects markers of both classical PPARγ transcriptional agonism ( aP2 ) and PPARγ-driven anti-diabetic effects that occur through blocking phosphorylation of PPARγ at Ser273 ( Adiponectin ). Concurrent binding of endogenous and synthetic ligands Several endogenous PPARγ ligands have been identified that, similar to GW9662 and T0070907, covalently bind to Cys285 in the PPARγ LBP. These include the lipid 15-deoxy-Δ 12,14 -prostaglandin J2 (15d-PGJ2) and oxidized fatty acids such as 5-oxoeicosatetraenoic acid (5-oxoETE), 15-oxoETE and 9-oxooctadecadienoic acid (9-OxoODE) [24] , [25] , [26] . Synthetic antagonists covalently bind to PPARγ through a halogen exchange reaction [20] , whereas endogenous ligands covalently bind through a Michael addition [26] . We performed 19 F NMR to determine whether MRL20 can bind to the alternate site of PPARγ covalently bound to an endogenous ligand ( Fig. 7a ). Similar to studies with covalent antagonists, 19 F NMR shows that MRL20 binds to PPARγ covalently bound to one of several endogenous ligands. Alternate site binding to PPARγ bound to an endogenous ligand results in the appearance of a single 19 F MRL20 resonance with a chemical shift similar to the alternate site 19 F resonances populated when PPARγ binds two equivalents of MRL20 or when MRL20 binds to GW9662-PPARγ or T0070907-PPARγ. In the case of 15d-PGJ2, a lowly populated peak is observed corresponding to the chemical shift of MRL20 bound to the canonical LBP, which likely represents protein not completely modified by 15d-PGJ2 as previously observed [26] . 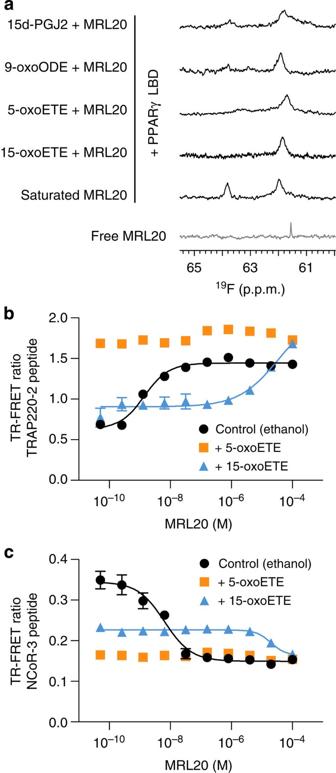Figure 7: Alternate site binding of MRL20 to PPARγbound to an endogenous ligand. (a)19F NMR analysis reveals that MRL20 binds to PPARγ LBD covalently bound to endogenous ligands. (b,c) TR-FRET assay demonstrates that alternate site MRL20 binding affects the interaction between (b) TRAP220-2 and (c) NCoR-3 for PPARγ LBD covalently bound to 15-oxoETE, but not 5-oxoETE. PPARγ LBD protein not covalently bound to an endogenous ligand but exposed to vehicle (ethanol) was used as a control; performed in duplicate, plotted as the average (±s.d.), and fit to a sigmoidal dose response curve. Figure 7: Alternate site binding of MRL20 to PPAR γ bound to an endogenous ligand. ( a ) 19 F NMR analysis reveals that MRL20 binds to PPARγ LBD covalently bound to endogenous ligands. ( b , c ) TR-FRET assay demonstrates that alternate site MRL20 binding affects the interaction between ( b ) TRAP220-2 and ( c ) NCoR-3 for PPARγ LBD covalently bound to 15-oxoETE, but not 5-oxoETE. PPARγ LBD protein not covalently bound to an endogenous ligand but exposed to vehicle (ethanol) was used as a control; performed in duplicate, plotted as the average (±s.d. ), and fit to a sigmoidal dose response curve. Full size image We performed a TR-FRET coregulator-binding assay to determine whether alternate site binding of MRL20 to PPARγ covalently bound to an oxidized fatty acid can affect coregulator interaction. Covalent attachment of 5-oxoETE, but not 15-oxoETE, significantly increases basal binding of TRAP220 peptide to PPARγ ( Fig. 7b ), and both endogenous ligands decrease the basal binding of NCoR peptide ( Fig. 7c ). This indicates that 5-oxoETE, but not 15-oxoETE, may impart significant AF-2 stabilization upon binding to PPARγ. This is consistent with the likely binding modes of 5-oxoETE and 15-oxoETE in the PPARγ LBP ( Supplementary Fig. 7 ). Addition of MRL20 to 5-oxoETE bound PPARγ did not affect coregulator recruitment, likely because the AF-2 surface is already maximally stabilized by 5-oxoETE as indicated by robust TRAP220 recruitment to 5-oxoETE-bound PPARγ. In contrast, MRL20 increased TRAP220 binding and decreased NCoR binding to 15-oxoETE bound PPARγ ( ∼ 20–30 μM EC 50 ). Thus, 15-oxoETE-bound PPARγ resembles apo PPARγ in terms of TRAP220 and NCoR binding, and therefore alternate site binding of MRL20 can impart significant additional stabilization of the PPARγ AF-2 surface and significantly affect coregulator peptide recruitment. The glitazones were first discovered using phenotypic screens to look for small molecules with anti-diabetic efficacy, and it was only later discovered that they activate PPARγ [27] . Subsequent studies using crystallography [28] or competitive ligand-binding assays revealed that these synthetic ligands and others bind to the canonical LBP of PPARγ, a variable-sized pocket within the interior of LBD conserved across the NR superfamily. Around the same time, the first identification of endogenous PPARγ ligands were made [29] , [30] , and more recent studies have revealed that endogenous ligands and synthetic ligands have overlapping binding sites in the PPARγ canonical LBP [24] , [26] , [31] , [32] , [33] . Thus, synthetic ligands are presumed to bind to PPARγ by competing with endogenous ligands for the same binding site. Our studies here demonstrate that PPARγ ligands can also bind to an alternate site and that this occurs via three pharmacologically relevant scenarios discussed below. First, alternate site binding can occur through binding two molar equivalents of the same ligand to PPARγ, one to the canonical LBP at high affinity and a second to the alternate site at a lower but potentially pharmacologically relevant affinity. This observation could affect the interpretation of studies examining the pharmacological function of PPARγ ligands. Although many PPARγ ligands bind to the canonical LBP with high affinity, often in the low nM range, in cell-based studies ligands are typically administrated at high pharmacological concentrations that exceed their canonical LBP binding affinity ranging from 10 μM to 150 μM [34] . For in vivo animal model studies it is difficult to know a priori the tissue-specific ligand concentrations in mice dosed with ligand on the order of several hundred mg per kg several times a day over many months. In these cases, it is possible that ligand concentrations could be high enough to elicit an alternate site functional effect through binding a second ligand. Second, alternate site binding can also occur when the PPARγ LBP is ‘blocked’ by covalently binding synthetic antagonists. Our studies demonstrate that PPARγ-dependent activity could be expected for some ligands well below 10 μM in the presence of a covalent antagonist. This calls into question whether the activity of a PPARγ ligand should be classified as PPARγ-independent if it shows activity when co-administered with a covalent antagonist. The action of daidzein on PPARγ is thought to occur by an LBD-independent mechanism because it activated the receptor in the presence of T0070907 (ref. 35 ). However, our studies indicate that daidzein binds and functionally activates the PPARγ LBD when the LBP is blocked by a covalent antagonist. For some ligands, such as BVT.13 and nTZDpa, covalent antagonist coadministeration significantly enhances the ability of the ligand to increase coactivator binding to PPARγ ( Supplementary Fig. 4c,g ). Finally, we show for the first time that alternate site binding can occur when the canonical LBP is bound by an endogenous ligand. Although the physiological role of covalently binding endogenous PPARγ ligands is not completely clear [26] , our data suggest that the alternate site could be a target for allosteric modulators if PPARγ is occupied by covalently binding endogenous ligands. In this realm, anti-cancer efficacies of PPARγ ligands in cell models are reported to be 1,000–10,000-fold higher than the ligand’s canonical LBP binding affinity [36] , [37] , [38] , [39] . In fact, coadministration of covalent antagonist with another PPARγ ligand does not block the anti-cancer activity and in some cases has been shown to synergize [40] . A characteristic feature of cancer cells is their ability to enhance de novo fatty acid and lipid biosynthesis, which can increase the concentration of oxidized fatty acids via β-oxidation, which bind covalently to the PPARγ LBP [26] . Thus, it is tempting to speculate that the mechanism of action affording the anti-cancer activity of PPARγ ligands occurs through the alternate binding site. In addition, obese individuals display enhanced de novo fatty acid and lipid biosynthesis or increased bioavailability from dietary sources, increasing the probability of PPARγ occupancy by oxidized fatty acids. In scenarios such as these, the alternate site may be the only means to modulate the activity of PPARγ using synthetic ligands. Our structural data show that alternate site binding affects NMR chemical shifts and amide proton exchange via HDX (that is, affects the hydrogen bond network) of residues that compose the AF-2 surface, which indicates an effect on the AF-2 surface conformation. The functional impact of this second ligand-binding event may be more notable for non-full agonists, which do not robustly affect the AF-2 surface or coactivator recruitment through binding to the canonical LBP. Mechanistically, there is evidence of an allosteric network running from the Ω loop to H3 via F287, to H12 and the AF-2 surface [32] , which also comprises a region called the ‘H3 electrostatic cluster’ [41] . Ligand binding to the LBP can directly stabilize the H12/AF-2 surface through formation of hydrogen bonds with residues within a ‘H12 subpocket’ near the AF-2 surface, including Y473 and H449 ( Fig. 8 ). However, the stabilization induced by alternate site binding likely occurs through an indirect mechanism, perhaps via the H3 cluster. Our data also indicate that graded PPARγ agonists have higher affinity for the alternate site than full agonists. This may be because PPARγ full agonists form a hydrogen bond with a specific residue on H12, Tyr473, which is a major contributor to their binding energy. Graded PPARγ agonists do not typically hydrogen bond with Tyr473, but instead use other bonding features to bind to the hydrophobic PPARγ LBP with high affinity that may be more conducive for alternate site binding. Of note, our previous PPARγ HDX studies used a 10 × molar excess of ligand [10] , [11] , [12] , [13] , and thus observations made in these previous studies likely include a mixture of canonical LBP and alternate site binding effects. 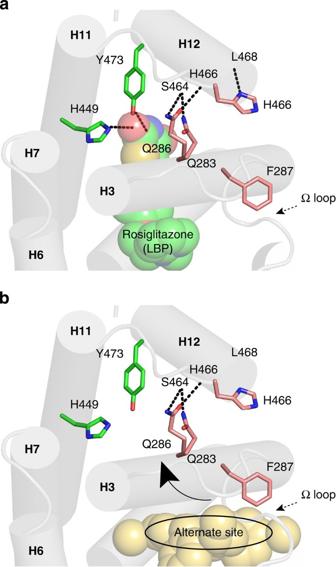Figure 8: Possible structural mechanism for indirect stabilization of the PPARγAF-2 surface via the alternate site. (a) Ligands such as rosiglitazone that bind to the PPARγ canonical LBP form hydrogen bonds with residues in the helix 12 pocket (Y473 and H449) to directly stabilize helix 12 and the AF-2 surface. (b) Ligands that bind to the alternate site may indirectly stabilize the AF-2 surface by stabilizing helix 3, facilitating hydrogen bond formation between side chains of residues on helix 3 to residues in the helix 11–12 loop, particularly in the presence of a bound coregulator, which could affect helix 12/AF-2 stabilization. Figure 8: Possible structural mechanism for indirect stabilization of the PPAR γ AF-2 surface via the alternate site. ( a ) Ligands such as rosiglitazone that bind to the PPARγ canonical LBP form hydrogen bonds with residues in the helix 12 pocket (Y473 and H449) to directly stabilize helix 12 and the AF-2 surface. ( b ) Ligands that bind to the alternate site may indirectly stabilize the AF-2 surface by stabilizing helix 3, facilitating hydrogen bond formation between side chains of residues on helix 3 to residues in the helix 11–12 loop, particularly in the presence of a bound coregulator, which could affect helix 12/AF-2 stabilization. Full size image Our work here extends several of our previous studies, including structure–function work revealing that PPARγ partial agonists display H12-independent activation mechanisms [12] , [13] . Data presented in these papers, performed at a 10 × excess of ligand, clearly show the involvement of regions of the ligand-binding pocket remote of AF-2, which we now know contains the alternate binding site. We have also shown that PPARγ ligands can affect PPARγ transcriptional activation and PPARγ-driven anti-diabetic efficacy through distinct mechanisms [10] , [11] . These latter studies addressed the paradox that exists for drugs that are anti-diabetic and activate PPARγ even though there are no loss-of-function mutations in the receptor of most type 2 diabetics. Phosphorylation of Ser273 (Ser273 ∼ P) represses the expression of a subset of PPARγ target genes, and full and partial agonists interfere with this post-translational modification to approximately the same degree. Blocking Ser273 ∼ P by ligands correlates more closely with the ability to increase the expression of adiponectin and other anti-diabetic effects than with the magnitude of transactivation of classical pro-adipogenic genes such as aP2. These observations suggest that a compound that binds and alters the level of Ser273-P independent of the degree of agonism of adipogenic genes can be anti-diabetic. We confirmed this in a subsequent report of SR1664, a compound that can block S273-P and is anti-diabetic even though it does not activate expression of adipogenic genes in cell culture and in obese mice [10] . We now show here that alternate site binding affects both classical PPARγ transcriptional agonism (increased receptor transactivation in a reporter assay and increased expression of aP2 ) and PPARγ driven anti-diabetic efficacy (increased expression of Adiponectin ) [10] , [11] . These observations indicate that the development of compounds that block PPARγ phosphorylation with little transcriptional activation can be complicated by alternate site binding. If alternate site binding contributes to the hyperactivation of PPARγ in vivo , where tissue/cell-specific drug concentrations are unknown, alternate site binding could explain why anti-diabetic partial agonists have not progressed to the clinic due to hints of side effects associated with full agonists and TZDs. This would make consideration of the alternate binding site critical to the development of a PPARγ modulator that only blocks Ser273-P without activating AF-2 regulated (for example, adipogenic) genes. Nearly all liganded PPARγ crystal structures have been solved with a single ligand bound to the canonical LBP. A crystal structure of PPARγ bound to a ligand at an alternate site would provide strong and direct evidence for the mechanism proposed in Fig. 8 . Despite our attempts, we were unable to obtain a co-crystal structure of MRL20 or MRL24 bound in the alternate site. However, a few published examples have revealed more complex structural mechanisms by which ligands bind to PPARγ’s large Y-shaped canonical LBP and the alternate site we identified here ( Fig. 9 ). A serotonin and a fatty acid metabolite can bind to distinct sub-regions in the canonical LBP [14] , and two non-covalently binding endogenous ligands have been crystalized within the PPARγ LBP [26] . However, in both of these cases, the ligands occupy a space within the canonical LBP similar to that of a single molecule of MRL20 bound in the LBP [13] and do not protrude out of the LBP near H3. Interestingly, the PPARγ partial agonist T2384 was crystalized with two molecules bound to one PPARγ. However, the authors did not explore the possibility that the alternate site T2384-binding event could affect function, this despite observing a bell-shaped response in a TR-FRET coregulator-binding assay with a high- and a low-affinity inflection point [42] . As mentioned above, the Ω loop has been implicated as part of an allosteric network that connects H3 to the AF-2 surface [32] , and our NMR studies as well as the T2384-bound PPARγ crystal structure [42] reveal that alternate site binding affects the conformation of the Ω loop. Our attempts to separate the independent functions of the canonical and alternate binding sites via mutagenesis were complicated because the mutant proteins behaved differently compared with wild-type PPARγ. Thus, we chose to use covalent antagonists to separate the function of the two sites by blocking binding to the canonical LBP, as they can be used as a pharmacological tool to study alternate site-binding in vitro and in vivo . 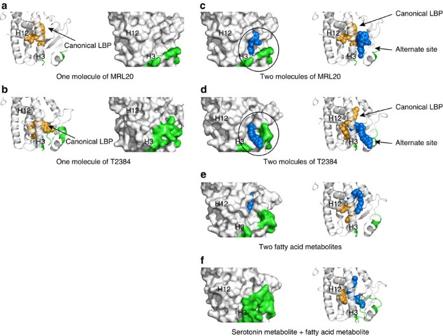Figure 9: Alternate site-bound ligands uniquely protrude around helix 3 to affect the conformation of the Ω loop. Ligands bound deep in the canonical LBP are coloured orange, and the second bound ligand, whether it occupies the alternate site region or not, are coloured blue; Ω loop region, if observed in the crystal structure, from M257-V277 is coloured green. Alternate site-bound ligands that affect the Ω loop conformation are also circled. (a) Co-crystal structure of the PPARγ LBD bound to one molecule of MRL20 (PDB: 2Q59). (b) Co-crystal structure of the PPARγ LBD bound to one molecule of T2384 (PDB: 3K8S; chain A). (c) Co-crystal structure of the PPARγ LBD with MRL20 (orange) (PDB: 2Q59) docked with a second MRL20 ligand (blue). (d) Co-crystal structure of the PPARγ LBD bound to two molecules of T2384 in the canonical LBP (orange) and alternate site (blue) (PDB: 3K8S; chain B). (e) Co-crystal structure of the PPARγ LBD bound to two molecules of 9-(S)-HODE (PDB: 2VSR). (f) Co-crystal structure of the PPARγ LBD bound to 5-methoxy-indole acetate (orange) and 15-oxoETE (blue) (PDB: 3ADW). Figure 9: Alternate site-bound ligands uniquely protrude around helix 3 to affect the conformation of the Ω loop. Ligands bound deep in the canonical LBP are coloured orange, and the second bound ligand, whether it occupies the alternate site region or not, are coloured blue; Ω loop region, if observed in the crystal structure, from M257-V277 is coloured green. Alternate site-bound ligands that affect the Ω loop conformation are also circled. ( a ) Co-crystal structure of the PPARγ LBD bound to one molecule of MRL20 (PDB: 2Q59). ( b ) Co-crystal structure of the PPARγ LBD bound to one molecule of T2384 (PDB: 3K8S; chain A). ( c ) Co-crystal structure of the PPARγ LBD with MRL20 (orange) (PDB: 2Q59) docked with a second MRL20 ligand (blue). ( d ) Co-crystal structure of the PPARγ LBD bound to two molecules of T2384 in the canonical LBP (orange) and alternate site (blue) (PDB: 3K8S; chain B). ( e ) Co-crystal structure of the PPARγ LBD bound to two molecules of 9-(S)-HODE (PDB: 2VSR). ( f ) Co-crystal structure of the PPARγ LBD bound to 5-methoxy-indole acetate (orange) and 15-oxoETE (blue) (PDB: 3ADW). Full size image The observation of alternate ligand-binding sites in general is relatively new in the NR field, and there is no general consensus on the importance of these sites. Though there is growing evidence to suggest that alternate binding sites are present in other NRs [43] , including ER [44] , [45] , [46] , AR [47] , [48] , [49] , TR [50] , [51] , [52] and VDR [53] , [54] , [55] , [56] , [57] , there is a lack of comprehensive studies to determine whether alternate site binding events can affect the structure and function of NRs. One main issue is how can alternate site ligand-binding events be detected? Most NR ligand-binding assays employ a ligand displacement assay, where a ligand that is radiolabelled or tagged with a fluorophore is competed with the ligand of interest. However, these displacement assays only report on the displacement of labelled ligand bound in the canonical LBP and will not generally detect an alternate site-binding event. As we demonstrate here, structural and biophysical assays can be employed to observe alternate site-binding events. In conclusion, our studies show that ligand binding to an alternate site can affect the structure and function of PPARγ. These observations reveal that ligand binding to PPARγ is not a simple competition between individual ligands and that the pharmacological properties of currently used synthetic PPARγ ligands are more complex than previously understood. Recognizing that this alternate binding site can affect PPARγ function may guide more informed development of a new generation of PPARγ drugs. Protein preparation and ligands PPARγ LBD (residues 203–477, isoform 1 numbering), full-length PPARγ (isoform 2, residues 1–505) and RXRα LBD (residues 223–462) were expressed in Escherichia coli BL21(DE3) cells as TEV-cleavable hexahistidine-tagged fusion proteins using protocols previously described [12] except that TCEP was used as a reducing agent. The final NMR buffer (Buffer C) consisted of 20 mM KPO 4 (pH 7.4) and 50 mM KCl. Ligands were either purchased from commercial sources or synthesized in-house based on prior reports [10] , [15] , [23] , [58] , [59] , including compounds 1 and 2 (Supplementary Figs. 8 and 9). Herein, references to structural studies use PPARγ1 sequence numbering, and references to functional studies use PPARγ2 numbering (Ser273 in γ2=Ser245 in γ1; Cys313 in γ2=Cys285 in γ1). NMR spectroscopy NMR was performed on 400 and 700 MHz ( 1 H frequency) Bruker NMR instruments at 298 K, calibrated using using an established relationship between the chemical shift difference of methanol-d 4 resonances and temperature [60] , equipped with a BBO or QNP probe (400 MHz) or BBO, TXI or QCI probe (700 MHz). Ligands were dissolved in DMSO-d 6 with the final sample concentrations containing<1% DMSO except in the 19 F observed titrations of MRL20 and MRL24 where direct addition of ligand to concentrated protein necessitated higher DMSO concentrations (<3%). Protein NMR and 19 F NMR (ligand-observe) experiments were performed as described previously [12] using pulse sequences provided with Bruker Topspin 3.0 and standard experimental parameters provided in Bruker Topspin 3.0 as well as methyl CHD 2 -detected experiments [61] . For quantitative comparison of relative 19 F NMR populations, a 10 s relaxation delay was used, otherwise 1 s delays were used. In addition to the raw value, corrected values for some titration points where free ligand is likely at or near maximum in Fig. 1 and Supplementary Fig. 1 were plotted. The correction was accomplished as follows. First, the signal from free ligand was subtracted, which was 0.44 (75 μM MRL24 solubility/171 μM PPARγ used) and 0.19 (30 μM MRL20 solubility/162 μM PPARγ used) canonical area units (signal from saturated canonical site) for MRL24 and MRL20, respectively. Second, the final titration point was re-run using a longer relaxation delay (10 s) and the relative change in area between the alternate site/free ligand signal and canonical site signal (due to different longitudinal relaxation rates) was determined and values were adjusted for these higher titration points as well (MRL20: 0.16 area units, MRL24: 0.2 area units). 19 F NMR calculation of alternate site-binding affinity The alternate site binding affinity using the relationship K D =([ L ][ R ])/[ LR ], where [ L ] and [ R ] are the concentration of free ligand and receptor and [ LR ] is the concentration of receptor bound to ligand. We assumed one additional binding site (two MRL20 molecules per PPARγ). The integral (area) of the 19 F NMR peaks indicates site occupancy [62] . 19 F NMR titration of MRL20 into buffer alone provided an estimate of 30 μM MRL20 solubility ( Supplementary Fig. 5 ), which is [ L ]. We saturated 330 μM PPARγ LBD with MRL20 and collected a 19 F NMR spectrum, which showed 89% occupancy of the alternate site compared with the canonical (after subtraction of signal from [ L ]). Occupancy of the alternate site decreases with a degree expected for the calculated K D upon dilution and re-concentration of PPARγ LBD. Definitions: [ LR ]=( I la / I ha )[ R 0 ]-[ L ]; [ R 0 ] is the overall protein concentration; I la and I ha are the integrals of the low- and high-affinity peaks, respectively; [ R ]=[ R 0 ]−[ LR ]; [ L ]=30 μM. Hydrogen/deuterium exchange mass spectrometry (HDX-MS) Solution-phase amide HDX experiments were carried out using a fully automated system [63] . Ten micromoles of His-PPARγ LBD protein (20 mM KPO 4 pH 7.4, 50 mM KCl) were pre-incubated with 1:2 molar excess of GW9662 at 4 °C overnight; this was the reference sample for HDX used to compare binding of MRL20. MRL20 was added at a 1:3 molar excess for 1 h. Five microlitres of protein solution were mixed with 20 μl of D 2 O-containing HDX buffer (20 mM KPO 4 , pH 7.4, 50 mM KCl) and incubated at 4 °C for 10, 30, 60, 900 and 3,600 s. Following on-exchange, unwanted forward or back exchange was minimized and the protein was denatured by dilution with 25 μl of quench solution (0.1% v / v TFA in 3 M urea). Samples were passed through an in-house prepared immobilized pepsin column [64] at 200 μl min −1 (0.1% v / v TFA, 15 °C) and the resulting peptides were trapped on a C 8 trap column (Hypersil Gold, Thermo Fisher). Bound peptides were gradient-eluted (5–50% CH 3 CN w / v and 0.3% w / v formic acid) across a 2 mm × 50 mm C 18 HPLC column (Hypersil Gold, Thermo Fisher) for 5 min at 4 °C. The eluted peptides were then subjected to electrospray ionization directly coupled to a high resolution Orbitrap mass spectrometer (Exactive, Thermo Fisher). Each HDX experiment was carried out in triplicate and the intensity weighted average m / z value (centroid) of each peptide isotopic envelope was calculated with in-house HDX Workbench software [65] . MRL20-induced changes in deuterium uptake were determined by subtracting average percentage deuterium uptake for 64 peptides spanning PPARγ LBD from the GW9662-PPARγ LBD sample and visualized with PyMOL (DeLano Scientific). Time-resolved Förster resonance energy transfer TR-FRET was measured using a PerkinElmer EnVision multilabel plate reader in 384-well plate format using peptides derived from the second LXXLL motif in the TRAP220 coactivator (TRAP220-2; residues 638–656; NTKNHPMLMNLLKDNPAQD) or the third CoRNR motif in the NCoR corepressor (NCoR-3; residues 2256–2278; DPASNLGLEDIIRKALMGSFDDK) containing a N-terminal FITC label with a six-carbon linker (Ahx); the C terminus was amidated for stability. Experiments contained 10 μl of protein mixture A: 50 nM hexahistidine-PPARγ LBD (or full-length PPARγ)+5 nM Anti-hexahistidine antibody labelled with Lumi4 Tb (Cisbio), 300–400 nM FITC-peptide (Lifetein) in TR-FRET buffer (0.1% BSA+Buffer C). Mixture A was plated, followed by the application of 10 μl of 2 × ligand or vehicle in TR-FRET buffer. Final concentration of DMSO (vehicle) was constant in all wells and <1%. The Lumi4–terbium donor was excited at 340 nm, its emission was monitored at 486 nm, and the acceptor FITC was measured at 520 nm. Fluorescence was measured after a 1–4 h incubation for PPARγ and then in some cases RXRα LBD+9- cis -retinoic acid was added and TR-FRET was measured again after a 4–12 h incubation. There was little change in signal in control wells where nothing was added during this second incubation. Plates were incubated at 4 °C and measured directly after removal from the cold in a room temperature instrument. In some cases, a gradual temperature-dependent reduction in the assay window occurred (for example, NCoR in the presence of GW9662) as the plate warmed during the longer plate readings. Ligand concentrations were varied in the direction of read (along rows and read along rows) when possible to minimize this effect within a ligand titration. Plates were also measured after equilibration at room temperature, which gave the same results. In some experiments, TR-FRET experiments were performed using biotinylated peptides for TRAP220 coactivator (TRAP220-2; residues 625-657; Biotin-KGGTPPPVSSMAGNTKNHPMLMNLLKDNPAQDF) and NCoR corepressor (NCoR-3; residues 2,250–2,283; Biotin-KGGFADPASNLGLEDIIRKALMGSFDDKVEDHG) with a streptavidin-d2 acceptor (CisBio). Ligand docking Ligand docking was performed using AutoDock Vina [66] using standard parameters with the degree of exhaustiveness set to 30. MRL20 was docked into the co-crystal structure of MRL20-PPARγ LBD (RCSB Protein Data Bank accession code 2Q59) or GW9662-PPARγ LBD (RCSB Protein Data Bank accession code 3B0R). Cell-based transactivation and gene expression 293T cells were batch cotransfected with Gal4-PPARg and UAS::luciferase reporter, plated, and after 18 h of incubation were treated with vehicle control (DMSO) or compound for 18 h. Luciferase activity was quantified 18 h after addition of compound with Britelite Plus (Perkin Elmer). For studies involving the covalent antagonist GW9662, before incubation with PPARγ ligands MRL20, MRL24 and rosiglitazone, cells were first pre-incubated with 5 μM GW9662 or vehicle control for 3 h. Jurkat T cells (ATCC TIB-152) were cultured in RPMI-1640 medium supplemented with 10% fetal bovine serum (FBS), 50 units per ml penicillin/streptomycin and plated at 5 × 10 5 cells (1 ml final volume). Cells were treated with ligand or vehicle control (DMSO) for 24 h and harvested for RNA isolation. NIH-3T3-L1 cells (provided by A. Chakraborty) were grown in DMEM media containing 10% fetal calf serum and 50 units per ml penicillin and streptomycin (Growth Medium). After 48 h, cells were switched to differentiation medium (Growth Medium with 1 μM dexamethasone, 0.5 mM isobutylmethylxanthine and 877 nM insulin but with 10% fetal bovine serum (FBS) instead of fetal calf serum) containing ligands or vehicle (DMSO) control. After another 48 h, cells were switched to a maintenance medium (Growth Medium with 877 nM insulin, also with FBS) containing ligands or vehicle control, and cells were harvested 3 days after inducing differentiation. Total RNA was isolated from cells using the RNAeasy kit (Qiagen). The RNA was reverse-transcribed using the iScript cDNA synthesis kit (Bio-Rad). Quantitative PCR reactions were performed with Faststart Universal SYBR Green Master (Roche) using an Applied Biosystems 9300 Real-Time PCR instrument with four biological replicates per condition. Relative mRNA expression was determined by the dd C t method normalized to GAPDH. Statistical analysis was performed using GraphPad Prism via one-way ANOVA with Tukey post hoc comparison of all treated conditions (NIH-3T3-L1 analysis) or Bonferroni post hoc comparison of selected conditions (Jurkat dose response analysis) using log transformed data. The sequences of primers used in this study are found in Supplementary Table 2 . How to cite this article: Hughes, T. S. et al . An alternate binding site for PPARγ ligands. Nat. Commun. 5:3571 doi: 10.1038/ncomms4571 (2014).